Molecular insights into genome-wide association studies of chronic kidney disease-defining traits Genome-wide association studies (GWAS) have identified >100 loci of chronic kidney disease-defining traits (CKD-dt). Molecular mechanisms underlying these associations remain elusive. Using 280 kidney transcriptomes and 9958 gene expression profiles from 44 non-renal tissues we uncover gene expression partners (eGenes) for 88.9% of CKD-dt GWAS loci. Through epigenomic chromatin segmentation analysis and variant effect prediction we annotate functional consequences to 74% of these loci. Our colocalisation analysis and Mendelian randomisation in >130,000 subjects demonstrate causal effects of three eGenes ( NAT8B , CASP9 and MUC1 ) on estimated glomerular filtration rate. We identify a common alternative splice variant in MUC1 (a gene responsible for rare Mendelian form of kidney disease) and observe increased renal expression of a specific MUC1 mRNA isoform as a plausible molecular mechanism of the GWAS association signal. These data highlight the variants and genes underpinning the associations uncovered in GWAS of CKD-dt. Chronic kidney disease (CKD) affects 10–15% of the population worldwide and is now recognised as the most rapidly increasing contributor to global burden of disease [1] , [2] . The costs related to CKD and end-stage renal disease (the terminal manifestation of CKD) are an enormous burden for all healthcare systems around the world [3] . The role of heritable factors in predisposition to CKD is well documented—our earlier family-based studies revealed high narrow-sense heritability for estimated glomerular filtration rate (eGFR) in two independent collections of European families [4] . These are consistent with a significant contribution of additive genetic factors to the overall variance in kidney function. The recent genome-wide association studies (GWAS) uncovered over 100 single-nucleotide polymorphisms (SNPs) associated with CKD-defining traits (CKD-dt: CKD, blood urea nitrogen, serum creatinine levels, eGFR and/or albuminuria) in the general population [5] , [6] , [7] . Some of the risk variants identified in these studies also predispose their carriers to the development of CKD in prospective case–control investigations [8] . Unfortunately, the biological mechanisms underlying the identified associations remain elusive as ≈90% of the genetic variants lie within non-coding DNA with no apparent function. Mechanistically, these variants do not act through the alteration of content/structure of the encoded messenger RNA (mRNA)/protein. Instead, they are more likely to exert their effects on the susceptibility to diseases through quantitative changes in gene expression, possibly largely in a tissue-specific manner. Indeed, these seemingly neutral variants appear to colocalise preferentially within chromosomal regions of regulatory importance for transcription and the variants associated with CKD-dt in GWAS show stronger enrichment for colocalisation to regulatory DNA in renal than non-renal cells [6] . These data suggest that variants associated with CKD-dt in GWAS may act through alterations of renal gene expression. Thus, human kidney tissue is essential to unravel the effects of these variants on the transcriptome. However, in contrast to other organs/tissues, large collections of human kidneys required for gene expression studies have not been widely available. For example, only 39 kidneys with full genome/transcriptome information are available in NIH-funded Genotype-Tissue Expression (GTEx) project [9] . This shortage of kidneys explains why a majority of functional gene expression analyses following GWAS for CKD-dt used mostly non-renal tissues or small collections of kidneys characterised by microarrays [5] , [10] . Unlike the latter, RNA-sequencing (RNA-seq) permits to refine transcriptome profiling by capturing all expressed transcripts directly without any a priori annotation [11] , [12] . RNA-seq is also more accurate at quantification of low abundance transcripts including long non-coding RNAs (lncRNAs), which are generally poorly represented on traditional microarrays. The recent RNA-seq-based analysis of kidneys from Tissue Cancer Genome Atlas (TCGA) offered the first glimpse into the renal identity of target genes for a small number of variants associated with CKD-dt in GWAS [13] . Here, through the analysis of 280 kidney transcriptomes profiled by RNA-seq and genotyped at DNA-wide level, we uncover renal gene expression partners (eGenes) for 25.6% of SNPs associated with CKD-dt in previous GWAS. We further demonstrate that a majority of these eGenes are associated with CKD or kidney function. Through single-tissue and multi-tissue analyses conducted in 44 non-kidney tissues from GTEx, we assign eGenes to additional 63.3% of CKD-dt GWAS SNPs. We also provide at least one functional annotation in silico for 74% of CKD-dt GWAS SNPs, either directly or by proxy. Our colocalisation studies and Mendelian randomisation (MR) analysis show causal effects of renal expression of three kidney eGenes ( NAT8B , CASP9 , and MUC1 ) on eGFR. Additional studies focused on MUC1 (a gene responsible for medullary cystic kidney disease (MCKD) type 1) reveal that renal expression of alternatively spliced mRNA isoform of MUC1 may be the key biological mechanism behind the genetic association signal captured in previous GWAS of CKD-dt. Kidney cis -expression quantitative trait locus analysis We first conducted a separate cis -expression quantitative trait locus ( cis -eQTL) analysis using a total of 5,499,848 SNPs and 14,518 and 19,862 kidney genes from 180 and 100 kidney transcriptomes from the TRANScriptome of renaL humAn TissuE (TRANSLATE) study [14] , [15] and The Cancer Genome Atlas (TCGA) [16] , respectively (Fig. 1a ). 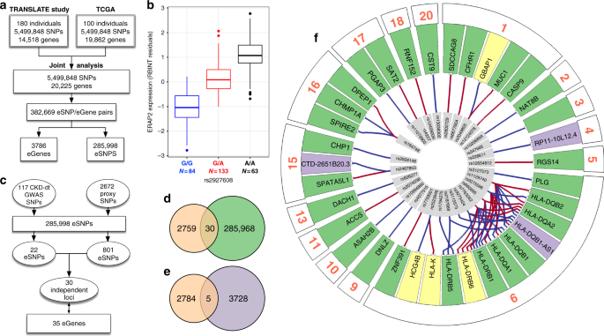Fig. 1 Cis-expression quantitative trait locus (cis-eQTL) analysis in human kidney.aStudy flow ofcis-eQTL meta-analysis. SNPs—single nucleotide polymorphisms, eSNPs—genetic variants with at least one renal expression partner eGene.bAssociation between rs2927608 genotype and renal expression ofERAP2—the most significant result fromcis-eQTL meta-analysis. RBINT—rank-based inverse normal transformation. The boxplot centre line shows the median, the two hinges show the upper and lower quartiles and the two whiskers show 1.5 times the interquartile range above and below the upper and lower quartiles respectively.cFlowchart showing the overlap between 117 variants associated with CKD-dt in genome-wide association studies (CKD-dt GWAS SNPs), their statistical proxies (linkage disequilibrium,r2>0.8) and kidney eSNPs (variants with at least one renal expression partner eGene).dVenn diagram—overlap between CKD-dt GWAS SNPs plus proxies (orange) and kidney eSNPs (green).eVenn diagram—overlap between CKD-dt GWAS SNPs plus proxies (orange) and kidney best eSNPs (purple).fCircular representation of findings fromcis-eQTL analysis for variants identified CKD-dt GWAS. eGenes are ordered radially by genomic and chromosomal location, coloured by gene biotype (green—protein coding, purple—long non-coding, yellow—pseudogene) and labelled by their HUGO symbol. eGenes are connected to their eSNPs by lines whose colours are determined by the direction of gene expression change by GWAS CKD-dt risk allele (red—increase, blue—decrease). dbSNP reference cluster IDs are shown for each eSNP The brief characteristics of recruited individuals are given in Supplementary Table 1 . We then combined a common panel of 5,499,848 genetic variants and up to 20,225 genes from 280 kidney transcriptomes in the joint analysis of both studies. This analysis revealed 382,669 significant eSNP–kidney gene pairs after a correction for multiple testing (Fig. 1a ). A total of 3786 unique renal eGenes (approximately 17.2% of all kidney genes) had at least one associated eSNP within a distance of 1 Mb after correction for multiple testing (Supplementary Data 1 , Fig. 1a ). Fig. 1 Cis -expression quantitative trait locus ( cis -eQTL) analysis in human kidney. a Study flow of cis -eQTL meta-analysis. SNPs—single nucleotide polymorphisms, eSNPs—genetic variants with at least one renal expression partner eGene. b Association between rs2927608 genotype and renal expression of ERAP2 —the most significant result from cis -eQTL meta-analysis. RBINT—rank-based inverse normal transformation. The boxplot centre line shows the median, the two hinges show the upper and lower quartiles and the two whiskers show 1.5 times the interquartile range above and below the upper and lower quartiles respectively. c Flowchart showing the overlap between 117 variants associated with CKD-dt in genome-wide association studies (CKD-dt GWAS SNPs), their statistical proxies (linkage disequilibrium, r 2 >0.8) and kidney eSNPs (variants with at least one renal expression partner eGene). d Venn diagram—overlap between CKD-dt GWAS SNPs plus proxies (orange) and kidney eSNPs (green). e Venn diagram—overlap between CKD-dt GWAS SNPs plus proxies (orange) and kidney best eSNPs (purple). f Circular representation of findings from cis -eQTL analysis for variants identified CKD-dt GWAS. eGenes are ordered radially by genomic and chromosomal location, coloured by gene biotype (green—protein coding, purple—long non-coding, yellow—pseudogene) and labelled by their HUGO symbol. eGenes are connected to their eSNPs by lines whose colours are determined by the direction of gene expression change by GWAS CKD-dt risk allele (red—increase, blue—decrease). dbSNP reference cluster IDs are shown for each eSNP Full size image We then quantified the extent to which the best eSNP can account for the renal expression of their partner eGenes. Similar to previous studies in other tissues [17] , we noted a wide range in the magnitude of the genetic effect on kidney expression. Indeed, the variance in eGene expression explained by the most significant eSNP varied from very significant (73.5% (rs12366— LINC01291 , P = 7.66 × 10 −31 )) to negligible (0.000042% (rs1483780— ALDH7A1 , P = 7.65 × 10 −7 )). For the most significant protein-coding renal eGene ( ERAP2 ), the best eSNP (rs2927608) accounted for 60.8% variance in its renal expression ( P = 3.74 × 10 −304 , Fig. 1b ). To determine which of the eGenes have a kidney-enriched pattern of expression, we overlapped our collection of 3786 renal eGenes with those determined as having “tissue-specific” or “tissue-enriched” expression in the Human Protein Atlas (HPA) (Supplementary Data 2 ). We found over-representation for our eGenes within HPA kidney-enriched genes when compared to all other kidney genes identified in the dataset (25% (75/305), vs. 19% (3711/19,920), P = 0.0096 (Supplementary Data 2 )). Taken together, these data suggest that the abundance of almost one in five genes expressed in the kidney is under genetic control of common variants in - cis . We have also identified that renal eGenes are over-represented within HPA kidney-enriched genes. Kidney cis -eQTL analysis of CKD-dt GWAS SNPs We then sought to examine which variants associated with CKD-dt in GWAS (CKD-dt GWAS SNPs) are transcriptionally active in the kidney and uncover the identity of their partner renal genes. We identified 117 CKD-dt GWAS SNPs in publicly available resources (Fig. 1c , Supplementary Data 3 ). Of those, 30 (25.6%) overlapped ( r 2 >0.8) with our kidney eSNPs (Fig. 1d , Supplementary Data 4 ) and 5 (4.3%) with the best kidney eSNPs (Fig. 1e , Supplementary Data 4 ). A total of 35 renal genes were expression partners for CKD-dt GWAS SNPs (Supplementary Data 4 – 5 , Fig. 1c ). In total, 57 eSNP–eGene pairs were identified through an overlap analysis of CKD-dt GWAS SNPs with our eQTL catalogue. Some of CKD-dt GWAS eSNPs were associated with renal expression of more than one eGene; for example, rs7763262 was associated with seven renal genes (Fig. 1f ). Ten percent of the identified CKD-dt GWAS eGenes were either lncRNAs or pseudogenes (Fig. 1f ). For 26 (86.7%) CKD-dt GWAS eSNPs, the associated eGene was different from the closest gene (Supplementary Data 6 ). We next investigated whether CKD-dt GWAS SNPs are enriched for kidney eSNPs. This analysis showed 4.0-fold and 1.8-fold over-representation of kidney eSNPs amongst CKD-dt GWAS SNPs when compared to the matched sets of randomly selected autosomal SNPs or non-CKD-dt GWAS variants, respectively ( P = 1.60 × 10 −10 and P = 1.90 × 10 −3 ). We then investigated the cell-type specificity of the renal eGenes partnered with CKD-dt GWAS SNPs using single-cell RNA-seq database generated from three specimens of apparently normal human kidney secured after cancer nephrectomies [18] . Overall, we mapped 14 CKD-dt GWAS eGenes onto at least one of 14 separate cellular clusters; each corresponding to a different cell lineage (Supplementary Data 7 ). Several of the eGenes showed a ubiquitous pattern of abundance across renal cell clusters, while others were specific to one particular cellular lineages—that is, DPEP1 mapped exclusively to proximal tubule cells and TFDP2 was associated with cells of the ascending loop of Henle. These findings provide evidence for the key role of CKD-dt GWAS SNPs in regulation of gene expression in the kidney. By uncovering the identity of the expression partners of CKD-dt GWAS eSNPs, our results refine the association signals to specific targets within the locus and map them (where possible) onto the specific renal cell types. Kidney eGenes and renal phenotypes in Nephroseq Of the 35 renal eGenes, 29 were available for investigation in at least one of seven eligible gene expression datasets deposited in Nephroseq [19] . We explored associations between the renal expression of these genes and either case–control status (patients with kidney disease vs. controls) or eGFR in separate meta-analyses (Supplementary Data 8 – 9 ). Our analysis revealed that 13 (45%) and 16 (55%) of kidney eGenes were associated with kidney disease or eGFR after the correction for multiple testing in the absence of heterogeneity (Supplementary Data 8 – 9 ). A total of 20 (69%) eGenes were associated with at least one renal phenotype in Nephroseq. For 12 (41%) of these eGenes, the direction of association with renal phenotype(s) in Nephroseq was consistent with that expected from the allelic effects identified in GWAS and cis -eQTL analysis. For example, renal expression of SPATA5L1 showed positive association with CKD, consistent with the effect of CKD-detrimental allele of GWAS rs2467853 on the increased expression of this gene in our cis -eQTL studies (Fig. 1f ). In some cases, the Nephroseq analysis helped to narrow down the list of CKD-relevant targets. For example, of two renal eGenes associated with the same CKD-dt GWAS eSNP (rs2049805), only one ( MUC1 ) was associated with CKD and eGFR in Nephroseq. In summary, these data show that a majority of renal partner genes for CKD-dt GWAS eSNPs are associated with CKD or kidney function. cis -eQTL analysis of CKD-dt GWAS SNPs in other tissues We took advantage of transcriptome-wide information from 44 tissues in GTEx project to examine what proportion of the transcriptionally active CKD-dt GWAS SNPs is exclusive to the kidney. In addition, we exploited non-kidney cis -eQTL analyses to assign expression partners to CKD-dt GWAS SNPs without renal eGenes in our kidney discovery dataset. Of 30 CKD-dt GWAS eSNPs (and 1208 proxies), 28 (93%) also act as eSNPs in at least one non-renal GTEx tissue (Fig. 2a, b ). However, six of them are associated with different eGenes than those in the kidney (Fig. 2b ). For example, PLG is a partner to rs3127573 in the kidney, while in non-renal GTEx tissues, this variant is associated with the expression of SLC22A3 . Another CKD-dt GWAS eSNP (rs9275424) was associated with the same eGene ( HLA-DRB1 ) in the kidney and GTEx tissues but the direction of this association was different between renal and non-renal tissues. In total, nine eSNP–eGene pairs (15.8% CKD-dt GWAS eSNP–eGene pairs) appear as kidney-specific. Fig. 2 Tissue expression profiles of CKD-dt GWAS SNPs. a General overview of CKD-dt GWAS SNPs and their expression profiles in different tissues. b Detailed overview of CKD-dt GWAS SNPs in relation to presence (blue) or absence (grey) of eGenes across different tissues; kidney data are from the TRANSLATE study and TCGA, GTEx—Genotype-Tissue Expression project, eSNP—transcriptionally active single-nucleotide polymorphism; kidney specificity was defined as (i) exclusive presence of eGene in the kidney or (ii) exclusive presence of eGene–CKD-dt GWAS eSNP association in kidney tissue (yellow dbSNP rsID label) or (iii) difference in identity of eGene partner between the kidney and non-kidney tissues (red dbSNP rsID label) or (iv) difference in direction of association of CKD-dt GWAS SNP with eGene between kidney and non-kidney tissues (green dbSNP rsID label) Full size image Further single-tissue analysis in GTEx revealed that of 87 CKD-dt GWAS SNPs (and 1871 proxies) without evidence for kidney eGenes, 49 operate as eSNPs in at least one non-renal tissue partnering with 193 eGenes. Nine of these eSNPs have an expression partner in only one GTEx tissue, while 79 other eSNPs are associated with eGenes in more than one GTEx non-renal tissues (Fig. 2a, b , Supplementary Data 10 – 11 ). We then applied multiple tissue meta-analysis [20] to 38 CKD-dt GWAS SNPs (and their 546 proxies) without any evidence for eGenes in either the kidney of non-kidney single-tissue analyses. This approach identified 190 additional unique eSNP–eGene pairs covering 25 unique CKD-dt GWAS loci and 176 unique eGenes (Fig. 2a, b , Supplementary Data 12 ). Using PhenoScanner [21] we then compared kidney-specific and “ubiquitous” CKD-dt GWAS non-HLA eSNPs for association with non-CKD phenotypes from previous GWAS (Supplementary Data 13 ). 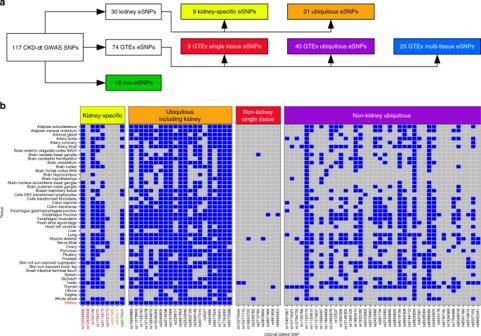Fig. 2 Tissue expression profiles of CKD-dt GWAS SNPs.aGeneral overview of CKD-dt GWAS SNPs and their expression profiles in different tissues.bDetailed overview of CKD-dt GWAS SNPs in relation to presence (blue) or absence (grey) of eGenes across different tissues; kidney data are from the TRANSLATE study and TCGA, GTEx—Genotype-Tissue Expression project, eSNP—transcriptionally active single-nucleotide polymorphism; kidney specificity was defined as (i) exclusive presence of eGene in the kidney or (ii) exclusive presence of eGene–CKD-dt GWAS eSNP association in kidney tissue (yellow dbSNP rsID label) or (iii) difference in identity of eGene partner between the kidney and non-kidney tissues (red dbSNP rsID label) or (iv) difference in direction of association of CKD-dt GWAS SNP with eGene between kidney and non-kidney tissues (green dbSNP rsID label) This analysis showed that significantly fewer kidney-specific variants were associated with non-CKD traits in GWAS when compared to “ubiquitous” CKD-dt GWAS non-HLA eSNPs, respectively ( P = 0.03, Supplementary Table 2 ). In summary, using single-tissue and multi-tissue analyses we showed that a vast majority (88.9%) of CKD-dt GWAS loci are transcriptionally active within renal and non-renal human tissues. We also showed that a significant proportion of the uncovered SNP–gene pairs is exclusive to the kidney and that kidney-specific subset of CKD-dt GWAS eSNPs is less likely to exhibit pleiotropic effects in GWAS when compared to “ubiquitous” CKD-dt GWAS eSNPs. Altogether, after these analyses, only 13 (11.1%) of CKD-dt GWAS loci were left without an expression partner eGene in any human tissue. In silico functional analysis of CKD-dt GWAS SNPs We used Ensembl variant effect predictor (VEP) [22] and newly derived adult kidney chromatin state segmentations (from ENCODE/Roadmap [23] Epigenomics raw data) of renal cells to functionally annotate all SNPs in each CKD-dt GWAS locus. We first determined that 19 of 117 sentinel CKD-dt GWAS SNPs variants (16%) mapped to exons across 22 overlapping genes, but only nine (8%) of these led to amino-acid changes in encoded proteins (Supplementary Data 14 ). Further analysis of 2672 proxies for CKD-dt GWAS SNPs identified 194 exonic variants, 22 of which led to amino-acid change (Supplementary Data 15 ). In total, 63 (54%) independent CKD-dt GWAS loci were classified as exonic either directly or by proxy (Supplementary Data 14 ) and 24 (21%) of these lead to an amino-acid substitution (with the remainder modifying sequence in untranslated exons or non-coding transcripts). Twenty two (19%) sentinel CKD-dt GWAS SNPs mapped onto regulatory DNA regions (either “transcription start site” or “enhancer” chromatin states) in adult human kidney tissue (Supplementary Data 14 ). In addition, three of them overlapped with a CpG island and one was localised directly in a transcription factor-binding site (Supplementary Data 14 ). The analysis of all proxies identified further 259 regulatory variants including 54 internal to CpG island, nine overlapping a transcription factor-binding site and 248 mapping onto either “transcription start site” or “enhancer” chromatin in adult human kidney tissue (Supplementary Data 15 ). In total, 69 (59%) independent CKD-dt GWAS loci showed evidence for a regulatory effect on gene expression either directly or by proxy. Of these, 23 (20%) showed no overlap with the VEP annotations (no evidence for exonic sequence modification). In summary, through the most comprehensive analysis of all known independent variants associated with CKD-dt in genome-wide scans, we uncovered at least one functional annotation for a vast majority (86 of 117 (74%)) of them, either directly or by proxy. These annotations provide an important additional support for the biological interpretation of the findings from GWAS (Supplementary Data 14 ). For some of the CKD-dt GWAS loci, this additional level of annotation may help to prioritise the variants within the same locus. For example, the sentinel rs9962915 variant in EPB41L3 gene and 40 out of its 41 proxies have no regulatory or coding implications. Only one proxy SNP (rs1785418) of rs9962915 maps onto a promoter region of highly transcriptionally active chromatin in renal cells (Supplementary Data 15 ). These data suggest that rs1785418 is the strongest functional driver of the association uncovered in GWAS. Colocalisation of CKD-dt GWAS SNPs and kidney cis -eQTLs We took advantage of access to individual level data from 280 kidney transcriptomes to calculate regulatory trait concordance (RTC) score for each of 26 CKD-dt GWAS non-HLA cis -eQTL signals. We chose to use RTC over Bayesian-based approaches (such as coloc ) [24] for several reasons. First, unlike coloc (that uses summary statistics), RTC makes full use of individual level data so that no information is lost unnecessarily [25] . Second, RTC is also known as generally more powerful in detecting colocalisation signals than coloc since it does not have to rely on the overlapping variants in both GWAS and eQTL datasets for analysis—a requirement that may reduce the chances of identifying significant results [25] . In addition, in the presence of multiple causal variants within a locus RTC shows greater accuracy (defined as the ratio of correctly predicted observations to the total observations) and recall rate (defined as the ratio of correctly predicted positive observations to the all actual positives) than coloc [24] . 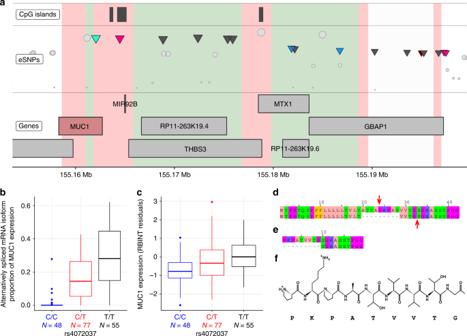Fig. 3 Functional analysis of MUC1.aFunctional annotations ofMUC1locus on chromosome 1. Top track—high-confidence CpG islands. Middle track—variants associated with the renal expression ofMUC1(MUC1eSNPs) represented as triangles and coloured by their functional consequences; blue—non-coding exonic, pink—mapping onto CpG islands, green—splice variant, grey—no annotations, the sentinel variant outlined in red, other tested eSNPs are shown as circles. The height of each eSNP is determined by the negative log10Pvalue for association withMUC1expression in the kidney, so that eSNPs more significantly associated withMUC1are higher than those less significantly associated. Bottom track—genes and a genomic scale bar for chromosome 1 in Mb. The coloured background reflects annotations from summarised chromatin states in adult human kidney tissue, red denotes transcription start site chromatin, green—transcribed chromatin, white—silent.bRenal expression of alternatively splicedMUC1mRNA isoform in the TRANSLATE study and TCGA. Data are standardised expression (means and standard errors) stratified on rs4072037 genotype. The boxplot centre line shows the median, the two hinges show the upper and lower quartiles and the two whiskers show 1.5 times the interquartile range above and below the upper and lower quartiles respectively.cRenal expression of totalMUC1in the TRANSLATE study and TCGA. Data are standardised expression (means and standard errors) stratified on rs4072037 genotype. The boxplot centre line shows the median, the two hinges show the upper and lower quartiles and the two whiskers show 1.5 times the interquartile range above and below the upper and lower quartiles respectively.dN-terminus of pairwise alignment of alternatively spliced (bottom) and reference (top) MUC1 protein isoforms. Red arrows point to the predicted cleavage sites.eN-terminus of pairwise alignment of alternatively spliced (bottom) and reference (top) MUC1 protein isoforms after signal peptide removal.fPrimary structure of the nine residues missing in the N-terminus of the alternatively spliced MUC1 isoform We found that seven out of 26 (27%) signals tagged the same causal variant (RTC ≥0.9)—the CKD and eQTL association mapped to the same SNP within these loci (Supplementary Table 3 ). In some cases, the colocalisation analysis highlighted which of the eGenes associated with the same eSNP was a more likely driver of the association with CKD-dt—that is, rs2049805 was linked to two different expression partners ( GBAP1 and MUC1 ), but only one of them passed the RTC threshold for colocalisation ( MUC1 ) (Supplementary Table 3 ). In other cases, the RTC-based analysis suggested that none of the expression partners of the CKD-dt GWAS eSNP (i.e. rs2467853) colocalised with the CKD-dt GWAS association signal. In summary, we demonstrate which of the loci have evidence of sharing the same causal variant between renal gene expression changes and the risk of CKD. MR analysis We then used cis -eQTL data from the TRANSLATE study and TCGA and GWAS summary data from CKDGen consortium [6] to robustly investigate whether the renal expression of seven eGenes (implicated in the colocalisation analysis) is causal to changes in eGFR. These MR studies demonstrated causal effects of expression of three kidney eGenes ( NAT8B , CASP9 , and MUC1 ) on eGFR in at least two out of three MR models (Supplementary Data 16 ). The most consistent MR evidence for causality was detected for renal expression of NAT8B and MUC1 (Supplementary Data 16 ). Collectively, the MR analyses uncovered the renal genes through which the genetic variants are most likely to act on the risk of CKD. Combined annotation-dependent depletion framework of MUC1 Given the insights from MR and the evidence for the role of MUC1 in kidney disease [26] , we have selected this gene as a target for further analyses. Of 16 variants in proximity to sentinel MUC1 variant (rs2049805), seven have functional annotations (Supplementary Data 15 , Fig. 3a ). Using Combined Annotation-Dependent Depletion (CADD) we calculated the functionality scores for all these variants to identify those with the highest biological likelihood of effect on MUC1 expression. The highest relative CADD scores were assigned to rs4072037 and rs12411216 (12.19 and 10.61, respectively) (Supplementary Table 4 ). These scores put rs4072037 in the top 6% and rs12411216 in the top 10% of most functionally significant SNPs in the human genome. Of these, rs12411216 maps onto the CpG island within the promoter region for MUC1 , while rs4072037 operates as an alternative splice site acceptor (Fig. 3a ). Fig. 3 Functional analysis of MUC1. a Functional annotations of MUC1 locus on chromosome 1. Top track—high-confidence CpG islands. Middle track—variants associated with the renal expression of MUC1 ( MUC1 eSNPs) represented as triangles and coloured by their functional consequences; blue—non-coding exonic, pink—mapping onto CpG islands, green—splice variant, grey—no annotations, the sentinel variant outlined in red, other tested eSNPs are shown as circles. The height of each eSNP is determined by the negative log 10 P value for association with MUC1 expression in the kidney, so that eSNPs more significantly associated with MUC1 are higher than those less significantly associated. Bottom track—genes and a genomic scale bar for chromosome 1 in Mb. The coloured background reflects annotations from summarised chromatin states in adult human kidney tissue, red denotes transcription start site chromatin, green—transcribed chromatin, white—silent. b Renal expression of alternatively spliced MUC1 mRNA isoform in the TRANSLATE study and TCGA. Data are standardised expression (means and standard errors) stratified on rs4072037 genotype. The boxplot centre line shows the median, the two hinges show the upper and lower quartiles and the two whiskers show 1.5 times the interquartile range above and below the upper and lower quartiles respectively. c Renal expression of total MUC1 in the TRANSLATE study and TCGA. Data are standardised expression (means and standard errors) stratified on rs4072037 genotype. The boxplot centre line shows the median, the two hinges show the upper and lower quartiles and the two whiskers show 1.5 times the interquartile range above and below the upper and lower quartiles respectively. d N-terminus of pairwise alignment of alternatively spliced (bottom) and reference (top) MUC1 protein isoforms. Red arrows point to the predicted cleavage sites. e N-terminus of pairwise alignment of alternatively spliced (bottom) and reference (top) MUC1 protein isoforms after signal peptide removal. f Primary structure of the nine residues missing in the N-terminus of the alternatively spliced MUC1 isoform Full size image Analysis of rs12411216 effect on MUC1 promoter methylation Given the role of hypermethylation of MUC1 promoter in its transcriptional repression shown in different cells and tissues [27] , we examined if rs12411216 may operate through this mechanism in the human kidney. We conducted genome-wide methylation analysis of 96 renal samples from the TRANSLATE study. A total of six CpG sites were identified within the CpG island overlaying the MUC1 promoter region. However, none of them showed association with rs12411216 genotype (Supplementary Table 5 ). There was also no correlation between renal methylation within either of these CpG sites and kidney expression of MUC1 (Supplementary Table 6 ). Thus, the effect of rs12411216 on promoter methylation is unlikely to mediate the association between CKD-dt GWAS variant and MUC1 expression in the kidney. Effect of rs4072037 on alternative splicing of kidney MUC1 Rs4072037 maps to exon 2 of MUC1 and the presence of its alternate allele (T) creates a novel exon boundary in MUC1 and a novel mRNA isoform [27] , [28] . To confirm the presence of this specific MUC1 mRNA isoform in the kidney, we examined the transcriptome of all the TRANSLATE study and TCGA kidneys at the transcript level. Amongst 10 MUC1 mRNAs identified in the kidney, the alternatively spliced isoform was the second most abundant on average (Supplementary Table 7 ). Our data confirmed that the expression of this isoform was heavily dependent on the genotype of rs4072037 (Fig. 3b ). Indeed, carriers of one and two copies of the alternate allele of this splice variant have intermediate and the highest expression levels of the alternatively spliced MUC1 isoform when compared to the reference genotype (almost non-existent expression levels) (Fig. 3b ). The total renal expression of the MUC1 gene and its alternatively spliced isoform showed similar associations with the genotype (Fig. 3b, c ). Most importantly, our follow-up MR analysis revealed that the expression of alternatively spliced MUC1 mRNA isoform is causally related to eGFR in a stronger manner than the total level of renal MUC1 (Supplementary Table 8 ). These data suggest that the rs4072037-driven allelic effect on expression of a specific MUC1 mRNA isoform may be the key biological mechanism behind the genetic association signal captured in previous GWAS. Computational analysis of MUC1 protein isoforms The alternatively spliced MUC1 mRNA differs from the reference renal transcript (ENST00000612778) only by a 27-nucleotide deletion. This in-frame indel results in the removal of nine amino acids in the translated peptide and occurs toward the end of the signal peptide region (which is responsible for directing mucin-1 to the extracellular matrix, Fig. 3d ). Bioinformatics analyses predicted that the signal peptide cleavage site shifts from a TTA|PK motif in the reference protein to VTG|SG in the alternatively spliced isoform (Fig. 3d, e ). Therefore, the N-terminal amino-acid sequence in the protein isoform arising from the alternatively spliced mRNA loses nine residues (PKPATVVTG, Fig. 3e ). Although neither of the protein isoforms have a defined secondary structure (they are eminently, long, unstructured peptides protruding from the cell membrane), the rigidity of proline might confer particular properties to the reference protein isoform (Fig. 3f ) that are lost in the alternatively spliced isoform. Both the reference and alternatively spliced protein isoforms contain all the common functional sites and domains expected in a MUC1 isoform. Over 100 variants associated with CKD-dt have been uncovered in large-scale genetic studies [6] , [7] , [13] , [29] . Yet, the biological mechanisms underlying the genetic susceptibility to CKD have remained elusive and the progress in clinical translation of the findings from GWAS has been slow. We have made the first steps to eliminate the existing knowledge gap between sequence and consequence by: (i) shedding light on the functional characteristics of CKD-dt GWAS variants, (ii) assigning their robust gene expression partners (eGenes), (iii) providing evidence for causality between some of the identified eGenes and CKD and (iv) illuminating the molecular mechanisms of genetically mediated susceptibility to CKD. A majority of GWAS usually report only the most apparent molecular consequences of the sentinel variants, that is, SNPs in coding exons leading to amino-acid changes of the encoded proteins. Those typically represent only 5–10% of signals in GWAS of complex traits. Through extensive functional annotations including both coding and non-coding exons, alternative splicing, transcription factor-binding sites, CpG islands and transcriptionally active chromatin states (such as enhancers and promoters) in cells of kidney origin, we uncovered at least one potential molecular consequence of DNA sequence variation for 74% of CKD-dt GWAS loci. Functionally, the strongest evidence for biological significance of a GWAS SNP is represented by the union of in silico annotations with a signature of transcriptional activity in the kidney—for example, several variants in linkage disequilibrium (LD) with rs10206899 CKD-dt GWAS on chromosome 2 not only act as eSNPs for NAT8B but also map to transcriptionally active enhancer regions in renal cells from Roadmap Epigenomics. However, due to LD, eQTL analyses—even when combined with regulatory annotations—are not always sufficient to nominate the strongest biological genetic variant as the driver of the detected association. Our cis -eQTL analyses have identified eGenes for variants in 89% of CKD-dt GWAS loci. The eGenes are the key component in the chain of molecular events triggered by a sequence variant and culminating in CKD. As such, they represent legitimate targets for further mechanistic studies and the development of diagnostic and therapeutic strategies. We anticipate that larger collections of samples and/or different strategies (i.e. trans -eQTL studies) will be necessary to uncover eGenes for the variants in the remaining 11% of CKD-dt GWAS loci. Most importantly, our project reassigned the SNP–gene relationships within the majority of CKD-dt GWAS loci from that based on SNP–gene proximity to justification by molecular biology [30] . GWAS automatically assigned their top SNPs to their closest protein-coding gene(s), yet a majority of these variants operate through different genes; commonly very distant to the original association signal [31] . It is becoming increasingly clear that DNA variants may regulate expression of remote genes through interactions facilitated by chromatin looping [32] . High-throughput chromosome conformation capture studies can illuminate how the regulatory sequence variants can be brought into physical contact with a linearly distant target (i.e. eGene). Such studies will be necessary to further the functional interpretation of CKD-dt GWAS findings. The existence of an overlap between GWAS and eQTL analyses does not automatically mean that the identified eGene is the driver of the association between the SNP and CKD. Indeed, several other molecular scenarios including linkage (whereby two separate variants in LD are independently linked to the GWAS and expression signal) and pleiotropy (whereby the same genetic variant is associated with the gene expression and the phenotype in an independent manner) are recognised consequences of the apparent union of signals from GWAS and eQTL analysis [33] . Our results are robust to the alternative explanations, with the causality being confirmed in more than one MR method and the analyses being immune to the presence of heterogeneity and pleiotropy. One of the most important deliveries of this project is the illumination of a molecular mechanism underlying an association between a common and functionally neutral variant on chromosome 1 (rs2049805) and several CKD-dt in a previous GWAS [34] . The GWAS signal was initially thought to operate through either MTX1 or GDA genes, none of which exhibits a particularly strong pathophysiological connection to the kidney [34] . Our cis -eQTL studies uncovered that two other genes within this locus ( GBAP1 and MUC1 ) act as the renal expression partners for the GWAS signal, but only one of them ( MUC1 ) is causally linked to the risk of CKD. MUC1 encodes a membrane-bound glycoprotein present on the apical surface of epithelial cells as a part of the mucosal barrier against exogenous insults [35] . Renal expression of MUC1 has been localised to the loop of Henle and the distal nephron (including the collecting ducts). Single rare autosomal dominant mutations in this gene are a known cause of MCKD type 1—a monogenic form of CKD presenting with renal cysts and a progressive drop of eGFR [36] . Our data uncovered that rs4072037 (one of the common variants in strong LD with the sentinel GWAS SNP) influences the renal expression of MUC1 through an alternative splicing mechanism. Indeed, acting as an alternative splice site acceptor, rs4072037 stimulates renal production of a MUC1 mRNA isoform with a 27-nucleotide deletion. Renal expression of this specific MUC1 isoform shows stronger causal relationship with the drop in eGFR than other MUC1 mRNAs or in fact total MUC1 expression. Further studies will be required to uncover the exact cellular mechanisms underpinning the association between CKD and the alternatively spliced isoform of MUC1 , but it is tempting to speculate that it may impair the physiological qualities of the mucus layer possibly through altering the physico-chemical properties of the N-terminal region of the isoform. Interestingly, a recent proteomic analysis of urine revealed that urinary excretion of MUC1 is associated with the risk of renal impairment in the general population [37] and that the diagnostic value of urinary MUC1 to predict eGFR decline was actually stronger than that of microalbuminuria [37] . We are aware of both certain limitations and strengths of our analysis. For example, to maximise the power of gene discovery we had to combine many available resources with transcriptome-derived information on the human kidney. In particular, gene expression-phenotype meta-analyses conducted in Nephroseq were based on data from several different studies and included patients with different aetiologies of CKD. This may have resulted in a degree of phenotypic heterogeneity impeding on our power to uncover genes of relevance to CKD. The development of large-scale resources integrating genotype information with renal gene expression profiles from populations with lower degree of phenotypic heterogeneity should help to refine existing and uncover new molecular mechanisms underlying the predisposition to CKD in the future. On the other hand, our study is based on the largest number of RNA-seq-derived transcriptomes of apparently normal human kidneys collected for a purpose of eGene discovery. This sample size may explain why the number of renal eGenes for CKD-dt GWAS SNPs identified by us is much larger (by approximately 4-fold) than in the previous report that used fewer than 100 kidneys [13] . The progress in CKD management has been hampered by the limited knowledge of its genetic mechanisms. Our study has contributed to the narrowing down of this research-practice gap by highlighting the specific genes whose tissue expression explains the genetic susceptibility to CKD uncovered by GWAS. Some of the uncovered kidney genes whose RNA or protein products are clinically measurable (i.e. MUC1 ) may become attractive targets for the development of future diagnostics, that is, to detect an early decline in kidney health prior to the irreversible drop in eGFR. GWAS signals and their eGenes are also promising targets for the development of future treatments. Indeed, pharmacological therapies informed by genomics are already available for patients with cancer/cardiovascular disease but not yet those with kidney disease. To this end, further omics-based analyses of the kidney could help to catalyse the conversion of the current treatment of CKD from the management largely based on its modifiable risk factors into tailored nephroprotection. Ethical compliance The studies adhered to the Declaration of Helsinki and were approved/ratified by the Bioethics Committees of the Medical University of Silesia (Katowice, Poland), Bioethics Committee of Karol Marcinkowski Medical University (Poznan, Poland), Ethics Committee of University of Leicester (Leicester, UK) and the University of Manchester Research Ethics Committee (Manchester, UK). Informed written consents were obtained from all individuals recruited into the TRANSLATE Study. For the deceased donors from TRANSLATE-T, the consent was obtained from the members of the family. General characteristics of the discovery populations The TRANSLATE study recruited patients diagnosed with unilateral non-invasive renal cancer, eligible for elective nephrectomy and with no apparent history of primary nephropathy [14] , [15] . Phenotyping included taking personal history (by the use of coded questionnaires), physiological measurements (including height, weight, waist circumference, blood pressure) and securing blood/urine samples for further biochemical/molecular analysis [14] , [15] . Small fragments of renal tissue were taken directly from the healthy (unaffected by cancer) pole of the kidney immediately after nephrectomy for further DNA/RNA extractions [14] , [15] and renal histology. A recent extension of the TRANSLATE study (TRANSLATE-T) conducted “zero time” pre-implantation biopsy from deceased donors’ kidneys prior to transplantation [38] . A needle biopsy samples were collected within 6–28 h since the extraction time (donation after brain death) [38] . The material from each kidney biopsy sample was then used for further molecular processing. Basic clinical information about the donors was collected from available hospital documentation. DNA was extracted from the frozen kidney samples (upon prior homogenisation) using Qiagen DNeasyBlood and Tissue Kit. The extracted DNA was hybridised to Infinium ® HumanCoreExome-24 beadchip array composed of 547,644 markers. Genotype calls were made using GenomeStudio. RNA was extracted from kidney samples immersed in RNAlater using RNeasy Kits (Qiagen). Upon checking of RNA purity and integrity, a total of 1 μg of kidney RNA was subjected to Illumina TruSeq RNA Sample Preparation protocol with poly-A selection. The TRANSLATE libraries were sequenced using either 100 bp reads (on an Illumina HiSeq 2000) or 75 bp paired-end reads (on an Illumina NextSeq or HiSeq 4000) producing an average of 31 million paired reads and 5.3 Gb per sample. TCGA is a National Institute of Health (NIH)-sponsored resource with tissue samples collected from over 10,000 individuals with cancer [39] . Apart from cancer specimen, TCGA collected neo-plastically unaffected sample from the removed organ (where appropriate). Similar to the TRANSLATE study, a sample from cancer-unaffected part of the kidney was secured after its surgical removal and used for RNA isolation and transcriptome profiling. These samples have been used as a source of information on normal kidney transcriptome in both our and others’ studies [13] , [15] . TCGA individuals have only basic demographic information (age, sex, ethnicity) available for analysis [40] . DNA was extracted from blood using QiAAmp Blood Midi Kit [40] , hybridised with probes on Affymetrix SNP 6.0 array composed of 906,600 probes; genotype calls were conducted using the Birdseed algorithm. TCGA genotype data were downloaded from the GDC Portal’s legacy archive. Five hundred and twenty three cases/files were identified using the following query criteria: “project name”—“TCGA”, “primary site”—“kidney”, “sample type”—“solid tissue normal”, “race”—“white”, “data category”—“simple nucleotide variation”, “data type”—“genotypes”, “experimental strategy”—“genotyping array” and “access”—“controlled”. We downloaded the data for 110 individuals who had matching RNA-seq data from normal kidney tissue. Kidney RNA was extracted from snap-frozen samples using a modification of the DNA/RNA AllPrep Kit (Qiagen). The mRNA libraries were sequenced with 50 bp reads on a HiSeq 2000 yielding an average of 80.6 million paired reads and 7.9 Gb per sample. We used the same set of quality control filters for genotyped markers in both the TRANSLATE study and TCGA. Variants were excluded if their genotyping rate was <95%, they mapped to Y or mitochondrial DNA or had ambiguous chromosomal location or violated Hardy–Weinberg equilibrium (HWE) ( P <0.001) or had minor allele frequency (MAF) <5%. In total, 272,343 variants passed the quality control criteria in the TRANSLATE study and 659,711 in TCGA. All individuals in both the TRANSLATE study and TCGA were subjected to the same set of quality control filters. Individuals were excluded if their genotype missing rate was >5%, their heterozygosity rate was outside ±3 standard deviations from the mean value, they failed cryptic relatedness test based on identity-by-descent (IBD), they had ancestry other than European or had discordant sex information. The genotype missing rate and the heterozygosity rate were calculated using plink . The analysis of cryptic relatedness based in IBD was conducted using king [41] . Individuals’ ancestry was determined using SNPWeights [42] and EIGENSTRAT [43] . Screening for inconsistency between declared and genetic sex was carried out using plink . Two individuals from the TRANSLATE study and seven from TCGA were excluded based on the above quality control filters. Genotype imputation was conducted using minimac3 algorithm with 1000 Genomes Project’s Phase 3 European population as the reference panel on Michigan Imputation Server. The total number of imputed variants was 47,100,201 in the TRANSLATE study and 47,101,134 in TCGA. The following post-imputation quality control criteria were applied to all imputed markers. We excluded variants mapping to the same genomic position, non-SNPs, variants with imputation coefficient R 2 <0.4, variants with MAF <5% or those violating HWE ( P <1 × 10 -6 ). Both MAF and HWE were calculated in each study separately based on data for individuals who passed genotype quality control and had matching transcriptome information. Supplementary Table 9 shows numbers of markers flagged for exclusion based on post-imputation quality control filters. A total of 5,760,291 and 5,892,571 survived post-imputation quality filters and 5,499,848 common SNPs were included in further analyses of the TRANSLATE study and TCGA, respectively. Genotype principal components were calculated using plink and only using genotyped data that passed all genotype quality control filters. In line with the GTEx project [9] , [44] , the top three principal components were used as independent variables in all downstream analyses (where appropriate). In the TRANSLATE study, the top three principal components accounted for 16% of variation in genotypes and in TCGA for 17%. Similar percentages were reported in the GTEx project. Processing of next-generation RNA-seq data All generated raw reads were stored in FASTQ format. The base call and read quality were evaluated using FastQC ( https://www.bioinformatics.babraham.ac.uk/projects/fastqc/ ). The input library complexity was assessed using RNA-SeQC. The pre-processing of reads for adapter trimming was conducted by Trimmomatic. The reads were then pseudoaligned to the GRCh38 Ensembl transcriptome reference (Ensembl release 83). Data were downloaded from the GDC Portal using the following query criteria: “project name”—“TCGA”, “primary site”—“kidney”, “sample type”—“solid tissue normal”, “race”—“white”, “data category”—“raw sequencing data”, “data type”—“aligned reads” and “experimental strategy”—“RNA-Seq”. In total, 112 cases/files were identified; 103 of them had matching array-based DNA information that passed all quality control filters. Renal expression was quantified in transcripts per million (TPM) at a transcript level using Kallisto. Transcript expression values were then summed to give gene-level expression values. A gene was selected for downstream analyses if its expression in at least 50% of kidney samples within each population/sequencing batch was >0.1 TPM. Genes not meeting the above threshold of expression criterion or those on sex chromosomes were excluded from further analyses. Prior to any analyses, all sequenced samples underwent quality control checks including: (i) number of total reads, (ii) D -statistic test (a measure of within tissue sample—sample correlation) [41] , (iii) sex compatibility check (consistency between the reported sex and gene expression sex—determined based on XIST and male-specific region of the Y-chromosome genes expression), (iv) verification of correct sample labelling based on comparing DNA base calls obtained from RNA-seq using GATK [45] and DNA genotype calls and (v) visual inspection of principal component plots of processed TPM data. In the TRANSLATE study, 22 samples were excluded because their D -statistic was <0.75. In TCGA, one sample was excluded because it did not pass sex compatibility check and two more samples because they appeared as outliers in principal component plots of processed TPM data. The final number of samples that passed all sample quality control filters and had matching genotype data was 180 in the TRANSLATE study and 100 in TCGA. After applying gene expression quality control filters, 14,518 renal genes were identified for further analyses in the TRANSLATE study and 19,862 in TCGA. Prior to any statistical analyses, a set of normalisation procedures was applied to gene expression data measured in TPM in both populations. First, robust quantile normalisation [46] across all samples was applied to the logarithm of TPM values with offset of one (the robust version of quantile normalisation uses medians rather than the means of empirical quantiles). Second, extreme outliers (observations with a residual three times interquartile range below/above the lower/upper quartile of the model residuals) at the gene level were identified using robust linear regression and replaced with imputed values from re-fitted models without outliers. Third, for each gene, the TPM values were normalised using rank-based inverse normal transformation [47] . Fourth, probabilistic estimation of expression residuals [48] (PEER) was used to estimate hidden factors in the expression data: 30 hidden factors for the TRANSLATE study and 15 for TCGA. The number of hidden factors was determined based on sample sizes as suggested in the GTEx project [9] , [44] . cis -eQTL analysis A total of 180 TRANSLATE study individuals and 100 subjects from TCGA were included in cis -eQTL analyses. Of 180 TRANSLATE study subjects, 14 were recruited into TRANSLATE-T. The TRANSLATE study and TCGA provided information on renal expression of 14,518 and 19,862 genes, respectively. For the purpose of cis -eQTL meta-analysis, we used 14,155 kidney genes common to both studies. Further 6070 genes passed all quality control filters in one dataset (either TRANSLATE or TCGA). The same panel of 5,499,848 SNPs passed all quality controls in both studies and was used consistently in all cis -eQTL analyses in both studies. For all genes, transcripts and variants we used GRCh37 coordinates in all downstream analyses. The eQTL analysis was conducted using linear regression models, where the association between the genotype dosage and the normalised gene expression was adjusted for age, sex, the top three genotype principal components from autosomal DNA, PEER-derived hidden factors (as specified above) and TRANSLATE/TRANSLATE-T indicator (source of kidney tissue: nephrectomy or biopsy). An SNP was included in analysis if it was located within 1 Mb from the nearest boundary of the gene. The eQTL analyses were conducted initially in each study separately. If a gene was present in kidneys from only one study, the final statistical estimates of association between the gene and its in- cis SNPs were derived from this study. For renal genes expressed in both studies, the nominal P -values for association between SNPs and gene expression were combined using weights based on inverse variances of study-specific effect estimates in fixed-effect meta-analysis. All eQTL analyses were carried out using MatrixEQTL R package [49] . The first level of multiple testing correction was computed for each gene separately based on its all in- cis SNPs and permutation test. A total of 2000 permutations were performed on each SNP–gene pair. At each permutation (i) gene expression values coupled with covariates (except genotype and principal components) were randomly arranged, (ii) the association between each gene and each of its cis -SNPs was re-estimated, (iii) the re-estimated P values of each gene–SNP pairs from the two studies were combined (where appropriate, i.e. for common genes for both studies as described above). For each gene, the smallest combined P value was recorded providing the empirical distribution of the smallest meta- P value for each gene. Then, the smallest meta- P value for each gene was adjusted based on the gene’s empirical distribution of the smallest meta- P values. Finally, the permutation-adjusted meta- P values (one for each gene) were used to calculate FDR using qvalue R package. Genes with q values <5% were defined as eGenes. To determine a set of SNPs that had a statistically significant association with the expression of their in- cis genes, we adopted the same strategy as the GTEx project [9] , [44] . First, a genome-wide empirical (permutation-adjusted) P value threshold, P t , was chosen as the permutation-adjusted P value for the gene whose q value was closest to 5%. Then, assuming that F i ( x ) is the empirical cumulative distribution function of the smallest meta- P value for the i th gene (estimated using permutations), the threshold for the nominal meta- P values for the i th gene was defined as \(P_{\mathrm{t},i} = F_i^{ - 1}\left( {P_{\mathrm{t}}} \right)\) , where \(F_i^{ - 1}\left( \cdot \right)\) is the inverse function of F i (·). Variants associated with CKD-dt in previous GWAS We took advantage of the catalogue of 107 independent SNPs implicated in GWAS of CKD-dt from Ko et al. [13] . We then identified further 10 SNPs associated with CKD-dt by searching GWAS catalogue and PubMed against the following criteria: (i) statistically significant ( P <5 × 10 −8 ) association with one of the following phenotypes; creatinine levels, eGFR, cystatin, blood urea nitrogen, urinary albumin–creatinine ratio, CKD, end-stage renal disease, nephropathy, proteinuria, (ii) r 2 <0.2 with the SNPs in the catalogue by Ko et al. [13] . Thus, a total of 117 independent CKD-dt GWAS SNPs together with 2672 statistical proxies ( r 2 >0.8) were available for our further analysis (Supplementary Tables 15 – 16 ). Kidney gene expression profiles in Nephroseq We used Nephroseq [19] —a web-based platform for integrative data mining of comprehensive renal disease gene expression datasets—as a resource for association analysis between 35 eGenes and CKD-dt. A total of 214 kidney samples from five eligible studies by Nakagawa et al. [50] (53 individuals—48 cases with CKD and five controls), Ju et al. [51] (52 individuals—21 CKD patients and 31 controls), Peterson et al. [52] (31 individuals—25 lupus nephritis patients and six controls), Reich et al. [53] (31 individuals—25 IgA nephropathy cases and six controls) and Berthier et al. [54] (47 individuals—32 lupus nephritis cases and 15 controls) were available for analysis of association between renal eGenes and qualitative CKD-dt (based on comparison of cases and controls). In each of these studies, CKD-dt cases had a different renal diagnosis including CKD [50] , [51] , lupus nephritis [52] , [53] , [54] or glomerulonephritis [53] . A total of 350 kidney samples from five eligible studies by Ju et al. [51] (186 samples), Sampson et al. [55] (49 samples), Reich et al. [53] (24 samples), Rodwell et al. [56] (69 samples) and Peterson et al. [52] (22 samples) were available for analysis of association between eGFR and eGenes. Rodwell et al. [56] samples were the only kidney tissues secured from patients without kidney disease. All gene expression profiles were originally generated in those studies using microarrays; the data were then deposited in and re-processed by Nephroseq to facilitate analyses of association between individual genes and different renal phenotypes. For each of 29 available genes we generated a quantitative measure of association with the renal outcome. For qualitative phenotypes, this was a fold-difference (log base 2) in gene expression between the cases (patients with kidney disease) and controls. In analysis of association between eGenes and eGFR, we used Pearson’s correlation coefficient. The measures of association were then meta-analysed across studies by Stouffer’s Z method (weighted based on sample size and the binomial distribution of P values [57] , respectively)—for CKD case–control studies and Olkin–Pratt fixed-effect meta-analysis approach [58] —for eGFR studies. The level of statistical significance from the meta-analysis was then corrected for multiple testing using Bonferroni adjustment. The corrected level of statistical significance was calculated at 0.0017. Heterogeneity was examined using Cochran’s Q test. Analyses in GTEx project This NIH-sponsored publicly available database brings together information from DNA analysis and RNA-seq-derived transcriptome-wide profiles of 53 normal human tissues collected from 544 post-mortem donors ( https://www.gtexportal.org/home/tissueSummaryPage , accessed 31 July 2017) [9] . For the purpose of cis -eQTL analysis, we selected data from 44 tissues (with a number of individual matching genotype-expression samples of at least 100) [9] . With only 32 samples, the kidney tissue was not available for this analysis. Basic demographic information (age, sex and ethnicity) was obtained directly from the GTEx portal. In total, we used information from 9958 samples from 44 tissues for several purposes. First, to identify kidney-specific eGenes we examined the overlap between eGenes identified in the discovery renal dataset with the set of eGenes identified for each of 44 non-renal tissues. The information for all statistically significant eSNP–eGene pairs identified in each tissue separately was obtained from GTEx cis -eQTL analysis (v7 release) [9] , [44] . Second, we used the same type of overlap analysis to examine what proportion of the transcriptionally active CKD-dt GWAS SNPs is exclusive to the kidney. We used all statistically significant eSNP–eGene pairs from cis -eQTL analysis [9] , [44] in v7 GTEx. These were obtained from the GTEx portal (data accessed October 2017). Briefly, cis -eQTLs were identified for each tissue using a window of 1 Mb upstream and downstream from each transcription start site with a significance threshold of 5% FDR. The cis -eQTL analysis was conducted using genotypes of variants with MAF >0.01 from whole-genome sequencing and expression values of genes with expression above 0.1TPM in 20% of samples per tissue and at least six reads in at least 20% of samples. Third, we adopted a recently developed method to identify significant eQTLs in collections of mixed tissues by combining the results at each SNP through meta-analysis of samples from different tissues. The method, RECOV [20] , was developed based on the RE2 meta-analysis framework [59] and uses a covariance matrix to explicitly model the correlation of an SNP effect on the same gene’s expression in multiple tissues. Specifically, RECOV development was motivated by the insight that the same SNP may have similar effect on the same gene in related tissues (which was not considered by the previous methods) [20] . Summary statistic (i.e. SNP effect and its variance) at each SNP in 44 tissues from GTEx eQTL analysis (v7 release) [9] was downloaded from GTEx portal (data accessed October 2017). The statistical significance of the identified eQTLs was assessed by meta- P values and those with Benjamini–Hochberg FDR <0.05 were considered as statistically significant. Functional annotations The 15-state chromatin segmentation in adult kidney tissue was calculated from ChIP-seq signal data for four different histone modifications (H3K4me1, H3K4me3, H3K36me3, H3K9me3) in adult kidney tissue from Roadmap Epigenomics GEO Series GSE19465 (data accessed September 2017). The input bed files were binarised (using the background input signal) and combined into a single chromatin state segmentation using ChromHMM [60] following the standard Roadmap Epigenomics protocol [23] for the 15-state segmentation. The 15-state model file from Roadmap ( http://egg2.wustl.edu/roadmap/web_portal/chr_state_learning.html#core_15state ), data accessed September 2017) was used for the final segmentation by ChromHMM. These data were used to provide functional context to kidney eSNPs and CKD-dt GWAS SNPs. Ensembl VEP Ensembl VEP GRCh37, release 90 ( http://grch37.ensembl.org/Homo_sapiens/Tools/VEP?db = core ) was used to quantify the proportion of CKD-dt GWAS SNPs (and their proxies) that lead to changes in the sequence of exons in both coding and non-coding transcripts. The functional annotations were obtained for each of the core SNPs and all statistical proxies and then summarised by each core SNP. The data were obtained directly from Ensembl GRCh37 (release 90) using the biomaRt R package. The hg19 CpG island track “cpgIslandExt” was downloaded from the UCSC table browser (accessed 9 February 2018). It contains all CpG islands in the human genome with a GC content >50%, length >200 bp and a ratio of observed CG dinucleotides to expected CG dinucleotides (as determined by the number of individual C and G nucleotides in the region) of >0.6. All CKD-dt GWAS SNPs (and their proxies) were converted to vcf format and uploaded to the CADD web server v1.3 (accessed 10 May 2018, http://cadd.gs.washington.edu ) for annotation and scoring. The generated scores should be interpreted as measures of biological significance of a given SNP. The outputs were ordered by the PHRED-scaled CADD score from largest to smallest. All PHRED-scaled scores and SNP summary information are provided in Supplementary Table 20 . Enrichment analyses We first tested whether the overlap between the kidney eSNPs and SNPs from GWAS of CKD-dt was greater when compared to an overlap between kidney eSNPs with random set of common autosomal SNPs. A total of 100 random sets of autosomal SNPs (and their proxies in LD at r 2 >0.8) were used as reference SNPs [61] . These sets were generated with SNPsnap using unique kidney eSNPs as the input. SNPs were matched for MAF, number of SNPs in LD (“LD buddies”), gene density and distance to the nearest gene, allowing for maximum deviation of ±10% for MAF and ±50% for the other three criteria. All matched sets were non-overlapping with the input variants. The 1000 Genomes Phase 3 European population was used as the genotype reference panel. The statistical significance was calculated using Fisher’s exact test. We tested whether kidney eSNPs are over-represented amongst GWAS CKD-associated SNPs when compared to non-CKD-dt GWAS SNPs. We searched NHGRI–EBI GWAS catalogue downloaded on 17 October 2017 (released 10 October 2017) as the source of information for GWAS SNPs. Entries with missing positional or OR/beta information were removed and the positions of the remaining entries were converted to hg19 with the Bioconductor BiomaRt R package. We identified 13,168 unique genetic variants significantly associated with a trait at genome-wide level ( P <5 × 10 −8 ). All SNPs associated with CKD-dt were removed and the remaining 12,984 GWAS non-CKD-dt SNPs (and their proxies in LD of r 2 >0.8) were used for enrichment analysis. The statistical significance of the enrichment analyses was calculated using Fisher’s exact test. We divided 53 CKD-dt GWAS non-HLA eSNPs into those with kidney-specific eGenes and those with non-exclusively renal eGenes (ubiquitous). We then examined each group for association with 408 non-CKD traits and phenotypes in previously conducted GWAS using Phenoscanner [21] . We used P <5 × 10 −8 as a threshold for identification of significantly associated phenotypes in GWAS. The statistical difference for over-representation amongst non-CKD-dt GWAS SNPs between both groups was examined using Fisher’s exact test. Colocalisation analysis Colocalisation between CKD-dt GWAS and kidney cis -eQTL signals was examined using the RTC [62] . In brief, given the abundance of cis -eQTLs in the human genome, the interval overlap only is not sufficient to claim that a GWAS SNP and a cis -eQTL SNP tag the same causal variant [25] , [62] . However, if the GWAS SNP and the cis -eQTL indeed tag the same causal variant, conditioning on the GWAS SNP in regression analysis is expected to remove any significant association of the cis -eQTL signal observed within the locus [63] . For all genes with a significant cis -eQTL in a given interval, RTC approach takes the residuals of the standard linear regressions of normalised expression values of the genes on the GWAS SNP, namely pseudo-phenotypes, to re-examine cis -eQTL regressions in each test interval. Each SNP is then ranked based on their corresponding P values in the regressions using pseudo-phenotypes—the higher P value the smaller the rank. We assessed the impact of correcting for the GWAS SNP effect on each of the SNPs in the tested interval, using the RTC score of each SNP (( N -rank)/ N , where N is the total number of the SNPs in the interval); the higher the rank the smaller the score. If the same functional variant is tagged by the GWAS SNP and the cis -eQTL SNP, one would expect a high impact of correction for the GWAS SNP effect, and thus, a high P value in the pseudo-phenotype regression and a small rank and a high RCT score [62] . In our analysis, individual level data from 180 TRANSLATE and 100 TCGA kidney transcriptomes were pooled together to calculate RTC scores for each of 26 CKD-dt GWAS non-HLA cis -eQTL signals. Each of the examined loci was defined based on recombination coldspots [63] and we used a RTC score ≥0.9 as indicative for the colocalisation signal. MR studies MR analyses were conducted to examine whether seven kidney eGenes implicated in colocalisation studies are causally related to changes in eGFR. Summary meta-analysis data for association between these SNPs and eGFR from 133,413 individuals was downloaded from the CKDGen Consortium [6] . Summary data for association between SNPs and gene expression was obtained from our cis -eQTL analysis conducted in the TRANSLATE study/TCGA. The most significant independent SNPs ( r 2 <0.2, P <0.08) associated with expression of eGenes were selected for the analyses as instruments. We used three MR methods (robust inverse variance-weighted (IVW) method, penalised weighted median method and robust MR-Egger regression) [64] to estimate the causal effect of gene expression on eGFR. These methods provide protection against failure of assumptions of instrumental variables. The robust IVW and penalised weighted median methods down-weight the contribution to the causal estimate of candidate instruments with heterogeneous ratio estimates. Robust MR-Egger regression allows for all instrumental variants to be invalid and provides robust estimate with robust regression [64] . We set the following criteria for the indication of positive finding of causality: causal effect estimates from at least two of the three robust methods must be significant after multiple testing corrections. Point estimates and standard errors were calculated for each method separately. Since SNP–gene expression associations were estimated using standardised gene expression, the MR estimates can be interpreted as the effect on eGFR per 1-SD increment in gene expression. As sensitivity analyses, MR-Egger regression was used to detect pleiotropy and heterogeneity. Bonferroni adjustment was used for multiple corrections and the significance level was calculated at 0.05/7 = 0.0071. MR and sensitivity analyses were implemented in the R package MendelianRandomization [65] . Kidney DNA methylation analysis To determine the pattern of 5-methylcytosine residues in kidney DNA, we used 96 TRANSLATE study renal DNA samples (750 ng). DNA underwent bisulphite conversion with the use of the Zymo EZ DNA Methylation Kit. The converted DNA samples (4 μL, at 50 ng μL −1 concentration) were then hybridised with the Illumina HumanMethylation450 BeadChip array. The arrays were processed through Illumina confocal laser scanning system and the extent of regional methylation was quantified in M values—the latter correspond to the ratio of methylated intensity to un-methylated intensity and have statistical advantage over commonly used β -values [66] . Out of 96 TRANSLATE study individuals whose kidney DNA was hybridised to HumanMethylation450 BeadChip array, two were excluded because of sex information inconsistency between DNA methylation data and the reported sex data. One individual was excluded because of missing clinical information. All remaining 93 samples had call rate (calculated based on detection P value threshold of 1 × 10 −16 ) of at least 98%. Out of the 485,512 probes, 15,311 probes were excluded due to a call rate below 95% (based on detection P value threshold of 1 × 10 −16 ). Eleven thousand six hundred and forty eight probes on X/Y chromosomes, 29,233 cross-reactive probes and 17,302 probes containing common SNPs (MAF ≥ 1%) were also excluded. This left 418,581 probes available for downstream analyses. DNA methylation data that passed the above quality control filters was processed using the “dasen” method from the wateRmelon R package [67] . Each consonant letter in “dasen” stands for a specific type of data normalisation: “d”— background adjustment by adding the offset between Type I and Type II probe intensities to Type I intensities, “s”— between-sample quantile normalisation applied to Type I and Type II probes separately and “n”—indicating no dye bias adjustment (the two vowels, “a” and “e”, were added by the authors for ease of pronunciation). In addition to the wateRmelon R package, the following R packages were used for pre-processing DNA methylation data: minfi29 and missMethyl. For the purpose of the MUC1 -focused analyses, we selected six CpG sites mapping to the promoter region of MUC1 . We examined an association between methylation at each of these sites and the genotype of rs12411216 under an additive model of inheritance using linear regression. This analysis was conducted in 93 TRANSLATE study individuals with matching DNA methylation data and array-based genotypes. The analysis of association between the extent of methylation at each of six MUC1 promoter CpG sites and renal expression of MUC1 was conducted using the same cis -eQTL gene expression values in 82 TRANSLATE study individuals with matching transcriptome and kidney methylome data. Quantification of transcript-specific abundance of MUC1 isoforms Transcript abundances were estimated by Kallisto [68] from all available kidney samples (180 from TRANSLATE study and 100 from TCGA) and input data used in the cis -eQTL analysis described above. Kallisto was run in a manner identical to the global cis -eQTL analysis except that a single additional transcript sequence ( ENST00000612778 with 27 bp of exon 2 removed) was added to the reference transcriptome. The edited transcript sequence was labelled as “ENST00000612778-as”. Total MUC1 gene expression was calculated as for the purpose of the global cis -eQTL analysis (the sum of all MUC1 mRNA TPM values in each sample). All transcript and gene expression values were transformed and normalised in a manner identical to the cis -eQTL analysis. Analysis of association between MUC1 mRNA isoforms and genotype was conducted under an additive model of inheritance by multiple regression whereby the renal abundance of each MUC1 isoform was a dependent variable, SNP genotype, age, sex, batch, technical hidden factors and three principal components were used as independent variables. Robust IVW method was used to examine if MUC1 isoforms are causally associated with eGFR. MR-Egger regression was used to detect pleiotropy and heterogeneity. Bonferroni adjustment was used to correct for multiple testing and the corrected level of significance was calculated at 0.05/11 = 0.0045 (adjusted for the number of all MUC1 isoforms and total MUC1 ). MR and sensitivity analyses were implemented in the R package MendelianRandomization [65] . Bioinformatic analysis of MUC1 isoforms The translated peptide sequence of the alternatively spliced MUC1 transcript was identified using the ExPaSy server ( https://web.expasy.org/translate/ ). This protein sequence was compared to isoform ENSP00000484824 reported in the Ensembl database, and isoform P15941-1 ( https://www.uniprot.org/uniprot/P15941 ) found in the UniProtKB database. The pairwise protein alignments were computed using the Needleman–Wunsch algorithm [69] with default parameters ( https://www.ebi.ac.uk/Tools/psa/emboss_needle/ ). Alignment of the N-terminal regions of each sequence are presented with amino acids coloured according to their physico-chemical properties [70] . Overall prediction of functional domains and motifs was performed with InterPro ( https://www.ebi.ac.uk/interpro/ ). Identification of signal peptides and transmembrane regions was completed with SignalP ( http://www.cbs.dtu.dk/services/SignalP/ ), TMHMM ( http://www.cbs.dtu.dk/services/TMHMM/ ), and TOPCONS ( http://topcons.cbr.su.se/pred/ ). NetSurfP was used to predict both the residue accessibility and the secondary structure of the peptides. The secondary structure predictions (including transmembrane regions and unstructured regions) were further confirmed with Quick2D ( https://toolkit.tuebingen.mpg.de/#/tools/quick2d ). The predicted positions of O-glycosylation and N-glycosylation sites were obtained from the UniProtKB entry P15941 . The primary structure of the polymorphic peptide region (differing between the reference transcript and the alternatively spliced transcript) was drawn with PepDraw ( http://pepdraw.com ). Reporting Summary Further information on research design is available in the Nature Research Reporting Summary linked to this article.